A cohesin–OCT4 complex mediatesSoxenhancers to prime an early embryonic lineage Short- and long-scales intra- and inter-chromosomal interactions are linked to gene transcription, but the molecular events underlying these structures and how they affect cell fate decision during embryonic development are poorly understood. One of the first embryonic cell fate decisions (that is, mesendoderm determination) is driven by the POU factor OCT4, acting in concert with the high-mobility group genes Sox-2 and Sox-17 . Here we report a chromatin-remodelling mechanism and enhancer function that mediate cell fate switching. OCT4 alters the higher-order chromatin structure at both Sox-2 and Sox-17 loci. OCT4 titrates out cohesin and switches the Sox-17 enhancer from a locked (within an inter-chromosomal Sox-2 enhancer/CCCTC-binding factor CTCF/cohesin loop) to an active (within an intra-chromosomal Sox-17 promoter/enhancer/cohesin loop) state. SALL4 concomitantly mobilizes the polycomb complexes at the Sox s loci. Thus, OCT4/SALL4-driven cohesin- and polycombs-mediated changes in higher-order chromatin structure mediate instruction of early cell fate in embryonic cells. An embryo develops from the fertilized egg up to organized tissues and organs by enacting step by step its repertoire of cell differentiation. An essential question remaining in developmental biology is how this process (that is, cell specification and determination [1] ) takes place. Appropriate and coordinated gene expression is essential to the cell specification process. This complex biological phenomenon is driven by co-regulated transcriptional, genetic and epigenetic mechanisms, including the formation of multiplexed transcription factories, DNA and histone modifications, as well as changes in chromatin structure. More than three decades ago, experiments in Drosophila [2] demonstrated that the genome is organised within a three-dimensional (3D) chromatin architecture. We now further know that the genome is arranged in higher-order conformations created by looped chromatin-DNA domains. Chromatin looping occurs both in cis and in trans , following intra- and inter-chromosomal interactions secured by cohesin [3] , [4] , [5] , [6] , and insulated from each other by insulators encompassing CTCF-binding sites. Intergenic and intragenic enhancers fold onto gene promoter regions and drive transcriptional processes in a cell- and tissue-specific manner [7] , [8] . The genome is thus mainly transcribed in a developmental stage and cell-type-specific manner [9] . Depending on the stage of cell differentiation, the cohesin complex participates in both insulating CTCF-dependent and activating CTCF-independent DNA loops. The cohesin complex is more specifically involved in the chromosomal interactions within intra-topological domains [10] . However, the role of these chromatin architecture dynamics in cell fate decisions during early development as well as the molecular events mediating such dynamics, have been minimally investigated. Recent pioneering studies reported a change in the topological structure of chromatin when T cells differentiate into specific lineages [11] and stem cells towards a neuronal progeny [12] . However, which and how transcription or other factor(s) trigger such a change has not been elucidated. Pluripotent embryonic stem cells (ESCs), derived from the inner cell mass of the blastocyst or the early epiblast, are capable of recapitulating the first steps of embryogenesis, including cardiogenesis [13] . There are several key early developmental events by which prospective heart cells are specified to adopt cardiac cell fate. One of the earliest events is the formation of the ‘mesendoderm’ and subsequent segregation of endoderm and mesoderm. A tight transcriptional network including OCT4, SOX-2, NANOG and their downstream gene and protein targets secure ESC pluripotency [14] . However, one of these factors, OCT4, also plays a critical role in early cell fate determination in a gene dosage-dependent manner both in mouse embryos and in ESCs [15] , [16] , [17] . Indeed, we reported that an increase in the level of expression of OCT4 in pluripotent ESCs either by nucleofection of a transgene or by challenging cells with the cardiogenic morphogen bone morphogenetic protein 2 (BMP2), a phenomenon that normally occurs during the early embryonic development, results in a switch of the POU transcription factor from the SOX-2 to the SOX-17 gene regulatory regions. This phenomenon directs cells towards a mesendodermal lineage, and ultimately commits them towards a cardiac fate [16] . These early sequential events are crucial to ensure normal cardiogenesis in vivo, as evidenced by specific cardiac defects observed in mouse embryos derived from OCT4-downregulated epiblasts [15] . A greater insight into the molecular mechanisms underlying these cell-specific transcriptional genetic and epigenetic events will improve our knowledge of embryonic cardiogenesis and embryonic cell fate specification in general. By the use of single and sequential chromatin immunoprecicipitation (ChIP) assays as well as of chromosome conformation capture (3C) assays performed on chromatin of ESC-derived mesendoderm, we discovered that OCT4 targets the cohesin complex, and changes the higher-order chromatin structure at Sox-2 and Sox-17 loci to direct the fate of ESCs towards mesendoderm and cardiac mesoderm. We further found that the spalt-like C2H2 zinc-finger transcription factor SALL4 represents a second mandatory OCT4 partner that, together with SOX-17, mediates the cardiogenic-specific function of OCT4. SALL4 recruits polycomb complexes to the Sox loci, facilitating changes in higher-order chromatin structure. Furthermore, our data uncover a dual function of a Sox enhancer that acts both in cis and in trans , as an activator and a repressor, respectively, thus providing a regulatory switch to direct cell fate decision towards a cardiovascular mesodermal lineage. Co-expression of OCT4/SOX-17/SALL4 in early mouse embryos To better define the pattern of expression of OCT4 in the embryo and to identify its putative targets/partners in the instructive OCT4/SOX-17 mesendodermal transcriptional pathway that commits embryonic cells towards cardiogenic mesoderm, we performed whole-mount immunostaining in mouse embryos at embryonic day (E) E7.5, a stage of development when the first cardiac progenitors are determined in the lateral posterior region [18] . We first observed co-expression of OCT4, SOX-17 and SALL4 in extraembryonic visceral endoderm ( Fig. 1a–d ). Using a Sox17 Cre/+ mouse bred with Rosa26 tDTomato females, we further confirmed that OCT4 and SALL4 were expressed in the SOX-17 + cell lineage ( Fig. 1d,e ). 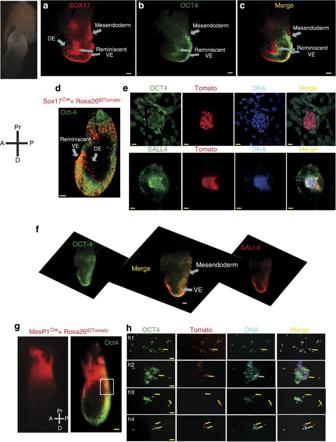Figure 1: Embryonic pattern of expression of SOX-17/OCT4/SALL4. Whole-mount staining of E7.5 mouse embryos with (a) anti-SOX-17- and alexa546-conjugated secondary antibody, (b) anti-OCT4- and alexa488-conjugated secondary antibody, (c) merged image (a,b). (d) Anti-OCT4 whole-mount immunostaining of E7.5 embryos derived from a Sox17cre/+breeder crossed with Rosa26tDTomatofemale. (e) the embryo proper was enzymatically dissociated and the cells were plated and fixed on coverslip. The cells were immunostained by an anti-OCT4 (upper panel) or anti-SALL4 antibody. Scale bars, 10 μm. Note that OCT4 is cytosolic in most of cells indicating a downregulation of the transcription factor. (f) Whole-mount staining of embryo using an anti-OCT4 and anti-SALL4 antibodies; a stack of images was acquired in confocal microscopy and reconstituted as a 3D image using AMIRA software. The merged image is shown in the centre. DE, definitive endoderm, VE visceral endoderm. (g) Anti-OCT4 immunostaining of E7.5 embryos derived from a MesP1cre/+breeder crossed with Rosa26tDTomatofemale. Whole-mount staining. (h) The posterior region of the embryo was enzymatically dissociated and cells were plated and immediately fixed on coverslip to be stained by an anti-OCT4 antibody and a secondary anti-alexa488 secondary antibody. Arrows indicate OCT4+ cells in the MesP1 cell lineage. OCT4 is either nuclear (h1) or cytosolic (h2, h3 and h4). Scale bars, 50 μm. Figure 1: Embryonic pattern of expression of SOX-17/OCT4/SALL4. Whole-mount staining of E7.5 mouse embryos with ( a ) anti-SOX-17- and alexa546-conjugated secondary antibody, ( b ) anti-OCT4- and alexa488-conjugated secondary antibody, ( c ) merged image ( a , b ). ( d ) Anti-OCT4 whole-mount immunostaining of E7.5 embryos derived from a Sox17 cre/+ breeder crossed with Rosa26 tDTomato female. ( e ) the embryo proper was enzymatically dissociated and the cells were plated and fixed on coverslip. The cells were immunostained by an anti-OCT4 (upper panel) or anti-SALL4 antibody. Scale bars, 10 μm. Note that OCT4 is cytosolic in most of cells indicating a downregulation of the transcription factor. ( f ) Whole-mount staining of embryo using an anti-OCT4 and anti-SALL4 antibodies; a stack of images was acquired in confocal microscopy and reconstituted as a 3D image using AMIRA software. The merged image is shown in the centre. DE, definitive endoderm, VE visceral endoderm. ( g ) Anti-OCT4 immunostaining of E7.5 embryos derived from a MesP1 cre/+ breeder crossed with Rosa26 tDTomato female. Whole-mount staining. ( h ) The posterior region of the embryo was enzymatically dissociated and cells were plated and immediately fixed on coverslip to be stained by an anti-OCT4 antibody and a secondary anti-alexa488 secondary antibody. Arrows indicate OCT4+ cells in the MesP1 cell lineage. OCT4 is either nuclear (h1) or cytosolic (h2, h3 and h4). Scale bars, 50 μm. Full size image OCT4 was also expressed together with SOX-17 and SALL4 in cells likely to be mesendodermal observed ingressing up and through the primitive streak ( Fig. 1f ). These mesendodermal cells further give rise to MesP1 + mesoderm, as revealed by the expression of OCT4 in cells of MesP1-derived lineage(s) in lateral plate mesoderm (LPM) in E7.5 embryos generated from a MesP1 cre/+ breeder crossed with Rosa 26 tDTomato females ( Fig. 1g,h ). SALL4 is an OCT4 target and partner in mesendodermal cells On the basis of our observations of the embryonic expression patterns of OCT4, SOX-17 and SALL4, we surmised that SALL4 could play a key role in the cardiogenic action of OCT4. To get more mechanistic insight into the role of SALL4, we used ESCs to generate a cell population enriched in mesendodermal cells. OCT4 is a common target of Nodal, BMP2 and Wnt signalling in ESCs [15] , [16] , [19] . We also reported that human ESCs (HUESCs) in which OCT4 expression was increased by twofold at the protein level [16] as observed in differentiating epiblast cells when compared with the inner cell mass [15] , recapitulated the early embryonic developmental process induced by the Nodal/BMP pathway [15] . Thus, we used OCT4 as an inducer of mesendoderm. Indeed, the HUESC population (OCT4OE) in which OCT4 was increased by 2.5-fold at the protein level (inset Fig. 2a ), expressed GOOSECOID MIXL1, HEX, SOX-17, SALL4, EOMES, BRACHYURY, SPARC and PDGFRα , but not ectodermal genes such as NESTIN, NOGGIN or PAX6 ( Fig. 2a ). SOX-2 and NANOG , two pluripotency genes, were markedly downregulated in this cell population. OCT4OE cells thus faithfully reflected a population referred to as mesendoderm. 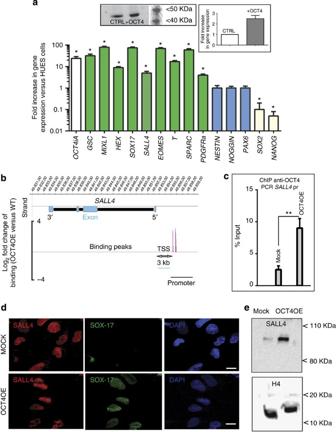Figure 2: OCT4 induces SALL4+/SOX-17+ mesendoderm by targeting SALL4 promoter. (a) OCT4 increase in expression gives rise to a mesendodermal cell population. OCT4-iA cDNA was nucleofected in HUESCs to increase by twofold the protein level of expression (inset: left panel: western blot anti-OCT4. Right panel: graphs representative of three gels, bands were quantified using Quantity one (Biorad) and normalized using actin as a housekeeping protein). Real-time PCR shows the fold increase or decrease in gene expression normalized to undifferentiated HUESCs ((mean±s.e.m., from four experiments, *Student’st-testP≤0.01). (b) OCT4-binding sites onSALL4promoter from ChIP-on-chip assay. Inset: ChIP–PCR anti-OCT4 from mock or OCT4OE cells. The result is represented as a fold change in occupancy in mesendodermal cells versus the undifferentiated HUESCs after normalization to the input sample. (c) OCT4 occupancy inSALL4promoter (pr) region was amplified by real-time quantitative PCR for mock or OCT4OE cells (mean±s.e.m., from three experiments, **Student’st-test,P≤0.01). (d) Oct4OE cells express both SALL4 and SOX-17. Mock (pcDNA nucleofected or Oct4OE cells were stained with anti-SALL4 and anti-SOX-17 antibodies and visualized at × 40 magnification by confocal microscopy. Scale bar, 10 μm. (e) Western blot anti-SALL4 of mock and Oct4OE cells. The histone H4 was used to normalize the blot. Figure 2: OCT4 induces SALL4+/SOX-17+ mesendoderm by targeting SALL4 promoter. ( a ) OCT4 increase in expression gives rise to a mesendodermal cell population. OCT4-iA cDNA was nucleofected in HUESCs to increase by twofold the protein level of expression (inset: left panel: western blot anti-OCT4. Right panel: graphs representative of three gels, bands were quantified using Quantity one (Biorad) and normalized using actin as a housekeeping protein). Real-time PCR shows the fold increase or decrease in gene expression normalized to undifferentiated HUESCs ((mean±s.e.m., from four experiments, *Student’s t -test P ≤0.01). ( b ) OCT4-binding sites on SALL4 promoter from ChIP-on-chip assay. Inset: ChIP–PCR anti-OCT4 from mock or OCT4OE cells. The result is represented as a fold change in occupancy in mesendodermal cells versus the undifferentiated HUESCs after normalization to the input sample. ( c ) OCT4 occupancy in SALL4 promoter (pr) region was amplified by real-time quantitative PCR for mock or OCT4OE cells (mean±s.e.m., from three experiments, **Student’s t -test, P ≤0.01). ( d ) Oct4OE cells express both SALL4 and SOX-17. Mock (pcDNA nucleofected or Oct4OE cells were stained with anti-SALL4 and anti-SOX-17 antibodies and visualized at × 40 magnification by confocal microscopy. Scale bar, 10 μm. ( e ) Western blot anti-SALL4 of mock and Oct4OE cells. The histone H4 was used to normalize the blot. Full size image ChIP-on-chip experiments, performed in both undifferentiated HUESCs and OCT4-induced mesendodermal cells, revealed that SALL4 was a major enriched target of OCT4 specifically in OCT4OE mesendodermal cells ( Supplementary Data set 1 ). The promoter region of SALL4 ( Fig. 2b ) was found highly occupied by OCT4 in OCT4-induced mesendodermal cells when compared with pluripotent HUESCs. ChIP–QPCR analysis confirmed the binding of OCT4 (fourfold enriched over the levels in mock cells) to the SALL4 promoter in OCT4-induced mesendodermal cells when compared with wild-type pluripotent ESCs (mock cells; Fig. 2c ). Immunostaining experiments showed that SALL4 expression was induced in OCT4OE mesendodermal cells compared with mock cells ( Fig. 2d ). Furthermore, SOX-17 expression was strongly induced in these OCT4OE cells compared with mock controls ( Fig. 2d ). Western blot analysis also showed an increase in the expression of SALL4 in OCT4OE mesendodermal cells ( Fig. 2e ). From these observations, we hypothesized that OCT4 and SALL4 cooperate to generate SOX-17 + mesendodermal cells. SALL4 mediates OCT4 switching from SOX-2 to SOX-17 promoters Next, we asked the question whether SALL4 was required for OCT4 switching between SOX-2A and SOX-17 3′ enhancers (see Supplementary Fig. 1 ), previously reported to be occupied by OCT4 (refs 16 , 20 , 21 , 22 ) as well as by H3K4me1 and p300 (refs 23 , 24 ) under different experimental conditions. To address this issue, we used a short hairpin RNA (ShRNA) silencing approach. Both immunofluorescence analysis and western blotting showed that nucleofection of HUESCs with a pSuper vector expressing a ShRNA targeting SALL4 successfully downregulated SALL4 protein, whereas SALL4 expression was unaffected in mock cells transfected with a scrambled ShRNA ( Fig. 3a ). Following SALL4 knockdown, ESCs maintained pluripotency, as shown by the normal expression of SOX-2 and NANOG ( Supplementary Fig. 2a ). This is consistent with the HUESCs being cultured on feeder layers, an experimental condition that maintains the undifferentiated state even in the absence of SALL4 (ref. 25 ). However, SALL4 knockdown resulted in OCT4 no longer being able to make the switch from the SOX-2A enhancer to the SOX-17 3′-enhancer in OCT4OE cells ( Fig. 3b ). It should be noted that OCT4 does not bind a 3′-region (region 2, R2, see Supplementary Fig. 1 ) of SOX-17 or the SOX2B [20] enhancer, both used as negative control regions ( Fig. 3b ). 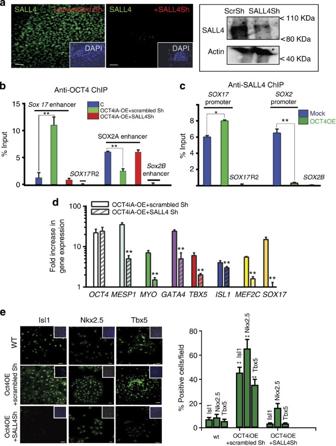Figure 3: SALL4 mediates the cardiogenic action of OCT4. (a) Anti-SALL4 immunofluorescence in mock (scrambled Sh-nucleofected cells) or SALL4Sh-nucleofected cells showed that SALL4 was downregulated in HUESC by nucleofection of a ShRNA. Scale bar, 50 μm. Right panel: western blot analysis of SALL4 in mock or SALL4Sh-transfected cells. (b,c) OCT4OE+scrambled Sh or OCT4OE+SALL4Sh-transfected cells were cultured on matrigel-coated dishes in the presence of FGF2- and MEF-conditioned medium for 4 days after nucleofection, to avoid interference of MEF chromatin in ChIP. (b) ChIP was performed using an anti-OCT4 antibody from mock (GFP nucleofected), OCT4OE+scrambled Sh cells or OCT4OE+SALL4Sh cells. PCR was performed using primers specific ofSOX-17orSOX-2enhancers A and B or matching a 3′-SOX-17R2 region (mean±s.e.m.,n=3; **Student’st-test,P≤0.01.). (c) Anti-SALL4 ChIP–PCR analysis ofSOX-17andSOX-2promoters.SOX17R2 andSOX2B enhancers were monitored to check the ChIP specificity. (d) Gene expression was monitored by real-time PCR in mock, OCT4OE cells or OCT4OE+SALL4Sh-transfected cells cultured on matrigel-coated dishes in the presence of FGF2- and MEF-conditioned medium for 4 days after nucleofection. Results are expressed as fold changes in OCT4OE cells versus undifferentiated HUESCs (mean±s.e.m.,n=3, **Student’st-testP≤0.01. (e) After 4 days post nucleofection, cells were dispersed with dispase and allowed to spontaneously aggregate to form EBs. Six days later, EBs were dissociated with trypsin, then plated for 14 h on fibronectin-coated labtech plates and proteins were visualized by immunofluorescence. The immunostained cells whose nuclei were labelled with DAPI were scanned with a BioRad confocal microscope. Background was set using undifferentiated HUESC stained with the same antibodies. Scale bar, 20 μm. Cells positive for the transcription factors were scored using DAPI as a reference to segment cells using Image J (right graph). The right graph shows statistical data (mean±s.e.m., from three experiments). **Student’st-test,P≤0.01. DAPI, 4,6-diamidino-2-phenylindole Figure 3: SALL4 mediates the cardiogenic action of OCT4. ( a ) Anti-SALL4 immunofluorescence in mock (scrambled Sh-nucleofected cells) or SALL4Sh-nucleofected cells showed that SALL4 was downregulated in HUESC by nucleofection of a ShRNA. Scale bar, 50 μm. Right panel: western blot analysis of SALL4 in mock or SALL4Sh-transfected cells. ( b , c ) OCT4OE+scrambled Sh or OCT4OE+SALL4Sh-transfected cells were cultured on matrigel-coated dishes in the presence of FGF2- and MEF-conditioned medium for 4 days after nucleofection, to avoid interference of MEF chromatin in ChIP. ( b ) ChIP was performed using an anti-OCT4 antibody from mock (GFP nucleofected), OCT4OE+scrambled Sh cells or OCT4OE+SALL4Sh cells. PCR was performed using primers specific of SOX-17 or SOX-2 enhancers A and B or matching a 3′- SOX-17 R2 region (mean±s.e.m., n =3; **Student’s t -test, P ≤0.01.). (c) Anti-SALL4 ChIP–PCR analysis of SOX-17 and SOX-2 promoters. SOX17 R2 and SOX2 B enhancers were monitored to check the ChIP specificity. ( d ) Gene expression was monitored by real-time PCR in mock, OCT4OE cells or OCT4OE+SALL4Sh-transfected cells cultured on matrigel-coated dishes in the presence of FGF2- and MEF-conditioned medium for 4 days after nucleofection. Results are expressed as fold changes in OCT4OE cells versus undifferentiated HUESCs (mean±s.e.m., n =3, **Student’s t -test P ≤0.01. ( e ) After 4 days post nucleofection, cells were dispersed with dispase and allowed to spontaneously aggregate to form EBs. Six days later, EBs were dissociated with trypsin, then plated for 14 h on fibronectin-coated labtech plates and proteins were visualized by immunofluorescence. The immunostained cells whose nuclei were labelled with DAPI were scanned with a BioRad confocal microscope. Background was set using undifferentiated HUESC stained with the same antibodies. Scale bar, 20 μm. Cells positive for the transcription factors were scored using DAPI as a reference to segment cells using Image J (right graph). The right graph shows statistical data (mean±s.e.m., from three experiments). **Student’s t -test, P ≤0.01. DAPI, 4,6-diamidino-2-phenylindole Full size image Interestingly, H3K27me3 and H3K4me3 epigenetic marks enriched on SOX-2 and SOX-17 promoter regions, respectively, in OCT4OE cells in the presence of SALL4 were not changed in the absence of SALL4 ( Supplementary Fig. 2b ), suggesting that SALL4 is critical to target histone-modifying enzymes to the SOX regulatory regions. To more specifically test the role of SALL4 in mediating OCT4-induced SOX-2/SOX-17 enhancer switching, we performed ChIP–PCR experiments on chromatin extracted from mock or OCT4-induced mesendodermal cells using an anti-SALL4 antibody, and interrogated the SOX-17 and SOX-2 promoters. SOX-17 promoter occupancy by SALL4 was significantly increased in OCT4-induced mesendodermal cells. In contrast, binding of SALL4 to the SOX-2 promoter was completely lost under the same experimental conditions ( Fig. 3c ). As observed for OCT4, SALL4 did not bind the Sox2B enhancer or the Sox-17 R2 region, confirming ChIP specificity. SALL4 was bound to a significant extent to the SOX-17 promoter in both OCT4OE and mock cells ( Fig. 3c ), occupied by trimethylated histone H3K27 in pluripotent cells ( Supplementary Fig. 2b ) in close proximity with trimethylated histone H3K4, confirming the bivalent state of the SOX-17 promoter [26] . We wondered whether this high occupancy of the SOX-17 enhancer by SALL4 was specific to HUESCs as they are more reminiscent of the epiblast stage rather than the inner cell mass stage of development. Furthermore, epiblast stem cells and naive ESCs feature some epigenomic differences [27] , [28] . We thus used a naive ESC line, namely the OCT4-inducible mouse CGR8 ESC clonal line, ZHBTc6, that we subcloned [15] from the parental line. Removal of tetracycline from the culture medium of these cells allows for a twofold increase in OCT4 expression ( Supplementary Fig. 3a ), a level of expression similar to the one reached in nodal- or BMP2-stimulated cells [15] . ChIP–PCR assays using chromatin extracted from induced or non-induced ZHBTc6 cells and an anti-OCT4 antibody showed that mouse OCT4 switched from the Sox-2C 3′-enhancer [20] to the Sox-17 3′-enhancer [21] , [22] ( Supplementary Fig. 3b,c ), as observed in HUESCs ( Fig. 3 ). OCT4 did not bind Sox2B enhancer in undifferentiated mouse ESC or the Sox17R2 region in OCT4-induced cells ( Supplementary Fig. 3b,c ). Intriguingly, as observed for OCT4, SALL4 also made this Sox promoter switch in induced CGR8 ZHBTc6 ESCs. In contrast to HUESCs, under basal conditions, SALL4 did not bind the Sox-17 promoter ( Supplementary Fig. 3c ). In the absence of SALL4 in short interfering RNA (siRNA) transfected and OCT4-induced mouse ESCs, OCT4 did not bind the Sox-17 enhancer, but remained on the Sox-2c enhancer ( Supplementary Fig. 3d ). This suggested that the occupancy of the SOX-17 enhancer by SALL4 in human ESCs might be related to their epiblast origin, and more heterogeneous status compared with naive mouse ESCs. SALL4 is required for the OCT4/SOX-17 cardiogenic pathway As OCT4 could not occupy the SOX-17 enhancer ( Fig. 3b ) and did not induce SOX-17 expression in the absence of SALL4 ( Fig. 3d ), we hypothesized that SALL4 was required for OCT4-mediated generation of cardiac progenitors. To address this question, we first monitored mesodermal and cardiac gene expression in OCT4-induced human mesendodermal and mesodermal cells and neighbouring cells in the presence or absence of SALL4. MESP1/2 , MYOCARDIN , GATA4 , TBX5 , ISL1 and MEF2C were induced by OCT4 upregulation in scrambled Sh-transfected cells, but were induced to a lower extent in the absence of SALL4 (that is, Sall4 Sh-transfected cells, Fig. 3d ). Cells nucleofected with OCT4 with or without SALL4Sh, or scrambled Sh, were allowed to spontaneously aggregate in suspension to form embryoid bodies (EBs) 4 days post nucleofection. Six days later, EBs were enzymatically dissociated and isolated cells plated on fibronectin-coated coverslips. Colonies of cardiac progenitors expressing ISL1, NKX2.5 and TBX5 appeared within 24-h following cell plating. Up to 50% of cells isolated from OCT4OE cell-derived EBs expressed these cardiac markers versus 10% of cells from mock EBs ( Fig. 3e ). EBs from cells overexpressing OCT4 with SALL4 knockdown generated very few cells expressing cardiac progenitor markers ( Fig. 3e ). Thus, SALL4 is required to mediate the cardiogenic function of OCT4. SALL4 recruits the polycomb complexes to the Sox loci SALL4 turns out to be a key target/partner in the OCT4-cardiogenic transcriptional pathway in both HUESCs and mouse ESC-derived mesendodermal cells. Hence, we chose to focus on the more naive mouse ESCs. To better understand its specific role, we investigated how SALL4 might act on the chromatin surrounding the Sox loci. Indeed, the histone modifications at the Sox loci did not occur in the SALL4 knockdown cells overexpressing OCT4 ( Supplementary Fig. 2 ). SALL4 targets many genes that are regulated in part by polycomb complexes and binds a protein of polycomb complex 1 (PRC1) [29] , [30] . We thus surmised that SALL4 recruited polycomb complexes to the Sox loci. We performed sequential ChIP assay in ZHBTc6 mouse cells, with or without induced OCT4 expression, first using an anti-SUZ12 or an anti-BMI1 antibody. The immunoprecipitated complex was detached from the anti-PRC antibodies by cleaving the IgG by dithiothreitol, washed and used in a second immunoprecipitation assay using an anti-SALL4 antibody. 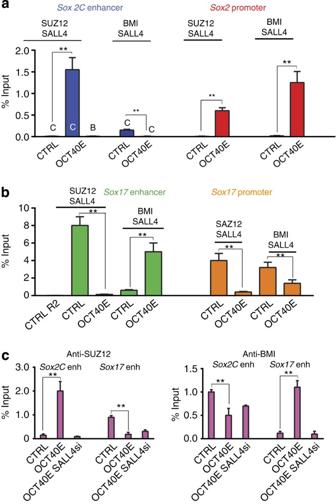Figure 4: SALL4 recruits the polycomb complexes PRC1 and PRC2 to theSox-2locus and the PRC1 complex to theSox-17locus. Sequential ChIP–PCR anti-SUZ12 or anti-BMI1 and then anti-SALL4 were performed from chromatin of control ZHBTc6 (+tetracyclin) ESCs (CTRL) or OCT4-overexpressing (ZHBTc6−tetracyclin) mesendodermal cells (Oct4OE). BothSox-2C(a) andSox-17(b) enhancers and promoters were interrogated.Sox2BandSox17R2regions were used as negative controls. (c) ChIP anti-SUZ12 (left panel) and anti-BMI (right panel) were performed from chromatin of control ZHBTc6 (+tetracyclin) ESCs (CTRL) or OCT4-overexpressing (ZHBTc6−tetracyclin) mesendodermal cells (Oct4OE). BothSox-2C andSox-17enhancers were interrogated. Data are expressed as mean±s.e.m., from three experiments, *Student’st-test,P≤0.01. Figure 4a shows that SALL4 specifically co-occupied, along with PRC2 (SUZ12), both the Sox-2C enhancer and Sox-2 promoter in mesendodermal cells following OCT4 upregulation. Interestingly, both PRC1 (BMI1) and PRC2 (SUZ12) were targeted to the Sox-2 promoter in the same cells, whereas BMI1 left the Sox-2C enhancer. Figure 4: SALL4 recruits the polycomb complexes PRC1 and PRC2 to the Sox-2 locus and the PRC1 complex to the Sox-17 locus. Sequential ChIP–PCR anti-SUZ12 or anti-BMI1 and then anti-SALL4 were performed from chromatin of control ZHBTc6 (+tetracyclin) ESCs (CTRL) or OCT4-overexpressing (ZHBTc6−tetracyclin) mesendodermal cells (Oct4OE). Both Sox-2C ( a ) and Sox-17 ( b ) enhancers and promoters were interrogated. Sox2B and Sox17R2 regions were used as negative controls. ( c ) ChIP anti-SUZ12 (left panel) and anti-BMI (right panel) were performed from chromatin of control ZHBTc6 (+tetracyclin) ESCs (CTRL) or OCT4-overexpressing (ZHBTc6−tetracyclin) mesendodermal cells (Oct4OE). Both Sox-2 C and Sox-17 enhancers were interrogated. Data are expressed as mean±s.e.m., from three experiments, *Student’s t -test, P ≤0.01. Full size image Both the Sox-17 3′-enhancer and promoter were enriched with PRC1 and PRC2 in control pluripotent cells. In mesendodermal cells, PRC1 and PRC2 occupation of Sox-17 promoter was significantly decreased. While PRC2 left Sox - 17 enhancer, PRC1 remained and even increased at this genomic region ( Fig. 4b ). The specific role of SALL4 as a polycomb recruiter was further tested by downregulating SALL4, while the OCT4 level of expression was concomitantly increased. Under this experimental situation, no recruitment of either PCR1 or PRC2 was observed on the Sox-2C enhancer. BMI was not recruited to the Sox-17 enhancer on OCT4 upregulation. SUZ12 could not be maintained on the Sox-17 enhancer in the absence of SALL4 ( Fig. 4c ). OCT4 changes chromatin architecture in mesendoderm formation SALL4 features double-chromatin-binding domains (DZF) [31] , [32] and recruits the polycomb complexes to the Sox loci ( Fig. 4 ), making it an ideal candidate to effect OCT4-mediated changes in chromatin structure. The cohesin complex plays a key role in organizing the 3D chromatin structure within topological domains [10] . We first tested whether the cohesin-loading protein NIPBL was required to mediate OCT4 switch from Sox-2C to Sox-17 enhancers. We thus designed experiments to limit the function of the cohesin complex under the cardiogenic action of OCT4. NIPBL was downregulated to 30% following transfection of ZHBTc6 cells with a siRNA versus mock cells transfected with a scrambled control siRNA ( Fig. 5a ). Expression of both OCT4 and NANOG was maintained in NIPBL-downregulated cells ( Fig. 5a inset). 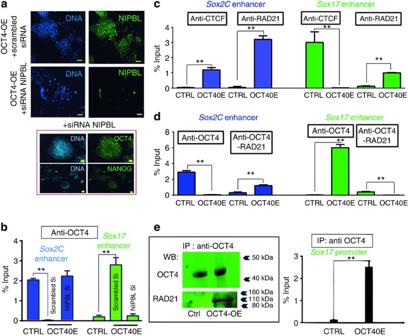Figure 5: RAD21- and CTCF-mediated OCT4-induced changes in the 3D configuration ofSox-17locus. (a) NIBPL was downregulated by a siRNA. Anti-NIPBL immunostaining of ZHBTc6 cells before differentiation within embryoid bodies of OCT4OE induced mesendodermal cells transfected with a scrambled siRNA or the NIPBL siRNA. Inset: OCT4 and NANOG expressions were found not affected in NIPBL-downregulated cells. Scale bar, 50 μm. (b) Anti-OCT4 ChIP was performed in control ESCs (CTRL) and OCT4-overexpressing mesendodermal cells (OCT4OE) in the presence or absence of NIPBL. Both theSox-2Cand theSox-17enhancers were interrogated. (c) Anti-CTCF and anti-RAD21 ChIP–PCR were performed from chromatin of control ZHBTc6 (+tetracyclin) ESCs (CTRL) or OCT4-overexpressing (ZHBTc6–tetracyclin) mesendodermal cells (Oct4OE). (d) Sequential ChIP–PCR anti-OCT4 and then anti-RAD21 were performed from chromatin of control ZHBTc6 ESCs (CTRL) or OCT4-overexpressing mesendodermal cells (OCT4OE). BothSox-2C(blue bars;c,d) andSox-17(green bars;c,d) enhancers were interrogated in real-time PCR. (e) Anti-OCT4 immunoprecipitation of whole cell extract from control (Ctrl) or OCT4-overexpressing mesendodermal cells (Oct4OE). The blot was incubated with both anti-OCT4 and anti-RAD21 antibodies. (f) Anti-OCT4 ChIP–PCR was performed from chromatin of control ZHBTc6 ESCs (Ctrl) or OCT4-overexpressing mesendodermal cells (Oct4OE).Sox-17 promoter was interrogated. Data are representative of three to four experiments (mean±s.e.m.). *Student’st-test,P≤0.01. Figure 5b shows that NIPBL siRNA transfected in pluripotent cells prevented OCT4 from relocating from the Sox-2C to Sox-17 3′-enhancer in OCT4OE mesendodermal cells. Figure 5: RAD21- and CTCF-mediated OCT4-induced changes in the 3D configuration of Sox-17 locus. ( a ) NIBPL was downregulated by a siRNA. Anti-NIPBL immunostaining of ZHBTc6 cells before differentiation within embryoid bodies of OCT4OE induced mesendodermal cells transfected with a scrambled siRNA or the NIPBL siRNA. Inset: OCT4 and NANOG expressions were found not affected in NIPBL-downregulated cells. Scale bar, 50 μm. ( b ) Anti-OCT4 ChIP was performed in control ESCs (CTRL) and OCT4-overexpressing mesendodermal cells (OCT4OE) in the presence or absence of NIPBL. Both the Sox-2C and the Sox-17 enhancers were interrogated. ( c ) Anti-CTCF and anti-RAD21 ChIP–PCR were performed from chromatin of control ZHBTc6 (+tetracyclin) ESCs (CTRL) or OCT4-overexpressing (ZHBTc6–tetracyclin) mesendodermal cells (Oct4OE). ( d ) Sequential ChIP–PCR anti-OCT4 and then anti-RAD21 were performed from chromatin of control ZHBTc6 ESCs (CTRL) or OCT4-overexpressing mesendodermal cells (OCT4OE). Both Sox-2C (blue bars; c , d ) and Sox-17 (green bars; c , d ) enhancers were interrogated in real-time PCR. ( e ) Anti-OCT4 immunoprecipitation of whole cell extract from control (Ctrl) or OCT4-overexpressing mesendodermal cells (Oct4OE). The blot was incubated with both anti-OCT4 and anti-RAD21 antibodies. ( f ) Anti-OCT4 ChIP–PCR was performed from chromatin of control ZHBTc6 ESCs (Ctrl) or OCT4-overexpressing mesendodermal cells (Oct4OE). Sox -17 promoter was interrogated. Data are representative of three to four experiments (mean±s.e.m.). *Student’s t -test, P ≤0.01. Full size image Then, we investigated the presence of cohesin component RAD21 and of CTCF at both Sox-2C and Sox-17 3′-enhancers in undifferentiated control mouse ZHBTc6 cells and OCT4-induced mesendodermal cells. Figure 5c shows that the Sox-2C enhancer was barely occupied by CTCF under control conditions, but was occupied to a much greater extent in OCT4-induced cells. In contrast, there was a pronounced loss of CTCF on the Sox-17 enhancer following OCT4 overexpression ( Fig. 5c ). RAD21 was bound to a low extent to the Sox-2C and Sox-17 3′-enhancers in the control cells, but bound both the Sox-2C and Sox-17 3′-enhancers in OCT4-induced cells ( Fig. 5c,d ). Sequential anti-OCT4/anti-RAD21 ChIP from chromatin extracted from OCT4-induced cells confirmed that both OCT4 and RAD21 were in the same transcriptional complex. These data also showed that in mesendodermal cells with an increased level of OCT4, RAD21 was removed from the Sox-17 3′-enhancer, while the cohesin component was loaded to the Sox-2C enhancer ( Fig. 5d ). These data are consistent with the Sox-2C enhancer on chromosome 3 interacting with the Sox-17 3′-enhancer on chromosome 1 in undifferentiated ESCs. This interaction was lost on OCT4 induction of mesendoderm. A similar OCT4/RAD21 complex switch was found in HUESCs and derived OCT4-induced mesendodernal cells ( Supplementary Fig. 4 ). Titration of cohesin by OCT4 was further suggested by a co-immunoprecipitation of RAD21 together with OCT4 in OCT4-overexpressing cells. RAD21 was barely detected in anti-OCT4 immunocomplex in control cells, but was recovered to a greater extent in OCT4-overexpressing mesendodernal cells ( Fig. 5e ). The formation of a new cohesin-dependent bridge between Sox-17 3′-enhancer and promoter was suggested by the binding of OCT4 on Sox-17 promoter in OCT4-induced mesendodermal cells ( Fig. 5f ). 3C is a suitable technique for looking at protein-mediated inter- and intra-chromosomal interactions. However, Sox-2C [20] and Sox-17 3′- enhancers [21] , [22] are close to their own promoters as expected for cohesin-regulated enhancers [33] , and are thus likely to be linked to the promoter [34] and active [35] . 3C could be unreliable to assess such short-range interactions [36] . We anyhow tried to use this technology to more specifically look at both inter- and intra-chromosomal interactions within the Sox-2 and Sox-17 loci and to further challenge the sequential ChIP–PCR data. Chromatin from control or OCT4-induced ZHBTc6 was enzymatically digested and religated from diluted chromatin. Using primers throughout the whole Sox-17 locus, including negative control primers hybridizing a Sox-17 exon or far 3′- untranslated genomic regions, we found that OCT4 specifically bound 3′- Sox-17 enhancer located 7.5 kb 3′of the promoter interacted with the promoter used as an anchor, suggesting that this enhancer was folded onto the Sox-17 promoter ( Fig. 6a ). We also looked at the 3D configuration of the Sox-2 locus. We observed the formation of a loop between the 5′- Sox-2A , as well as between the 3′- Sox-2C and the Sox-2 promoter used as an anchor in pluripotent stem cells. This finding is in line with the location of the cohesin complex on chromosomes 1 and 3 in cohesin Chromatin Interaction Analysis by Paired-End Tag Sequencing (Chia-PET) experiments [37] and with the previously identified Sox-2 enhancers [20] . Such loops were no longer observed in OCT4OE mesendodermal cells ( Fig. 6b ). 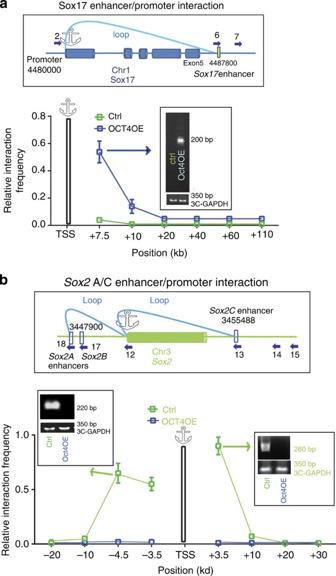Figure 6: OCT4 favours an enhancer/promoter loop within theSox-17locus and breaks aSox-2enhancer/promoter loop. 3C experiments were performed on digested and religated chromatin from undifferentiated ZHBTc6 cells or OCT4-induced mesendodermal cells. Primers spanning within theSox-2andSox-17loci and numbered as in Table 2 were used in PCR. Control primers such as in exons were used as controls (cartoons,a–c). The graphs show the frequency of interactions withinSoxloci on chromosomes 1 (a) or 3 (b) in both control (ZHBTc6 non-induced cells) and Oct4OE (ZHBTc6 induced) mesendodermal cells. Interactions frequencies were normalized using the GAPDH locus whose 3D configuration was assumed not to change, as GAPDH is expressed to the same extent in both pluripotent ESCs and OCT4OE (ZHBTc6 induced) mesendodermal cells. The relative interaction frequency value is thus set to one for the interaction measured between the control GAPDH fragments. Data are representative of four experiments (mean±s.e.m.). Figure 6: OCT4 favours an enhancer/promoter loop within the Sox-17 locus and breaks a Sox-2 enhancer/promoter loop. 3C experiments were performed on digested and religated chromatin from undifferentiated ZHBTc6 cells or OCT4-induced mesendodermal cells. Primers spanning within the Sox-2 and Sox-17 loci and numbered as in Table 2 were used in PCR. Control primers such as in exons were used as controls (cartoons, a – c ). The graphs show the frequency of interactions within Sox loci on chromosomes 1 ( a ) or 3 ( b ) in both control (ZHBTc6 non-induced cells) and Oct4OE (ZHBTc6 induced) mesendodermal cells. Interactions frequencies were normalized using the GAPDH locus whose 3D configuration was assumed not to change, as GAPDH is expressed to the same extent in both pluripotent ESCs and OCT4OE (ZHBTc6 induced) mesendodermal cells. The relative interaction frequency value is thus set to one for the interaction measured between the control GAPDH fragments. Data are representative of four experiments (mean±s.e.m.). Full size image Using primers matching the Sox-2C enhancer region used as an anchor and throughout the Sox-17 locus, we observed an interaction of chromosomes 3 and 1 harbouring the Sox-2 and Sox-17 genes, respectively. More specifically, such an inter-chromosomal interaction takes place in the regions encompassing the Sox-2C and Sox-17 3′-enhancers ( Fig. 7a ). This inter-chromosomal interaction was further confirmed by using 3D fluorescence in situ hybridization (FISH) analysis and probes mapping the Sox-2C and Sox-17 enhancers ( Fig. 7b ). In pluripotent stem cells, both alleles harbouring the Sox-2 and Sox-17 enhancer regions likely interacted within the chromosomal territory in nuclei in interphase. This interaction was lost in mesendodermal cells generated by OCT4 overexpression as observed in 3C assays and visualized in FISH experiments ( Fig. 7a,b ). 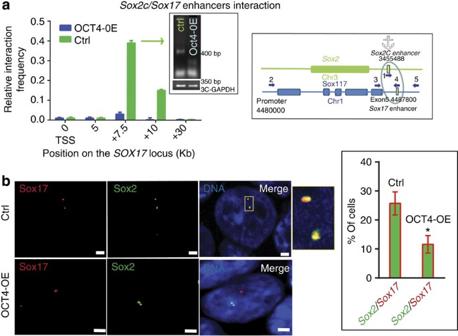Figure 7: OCT4 breaksSox-2/Sox-17enhancer inter-chromosomal interaction. (a) 3C experiments were performed on digested and religated chromatin from undifferentiated ZHBTc6 cells or OCT4-induced mesendodermal cells. Primers spanning within theSox-2andSox-17loci and numbered as in Table 2 were used in PCR. Control primers, such as in exons, were used as controls (cartoons,a–c). Interaction frequencies were normalized using the GAPDH locus. The graphs show the frequency of interactions between chromosomes (Chr) 1 and 3. The gels show the specificity of the amplicons of the peaks of interaction; the sequence of amplicons was checked by sequencing. The relative interaction frequency value is set to one for the interaction measured between the control GAPDH fragments. Data are representative of four experiments (mean±s.e.m.). (b) Illustration of FISH experiments using aSox2alexa488 andSox17alexa568 probes showing the interaction between chromosomes 1 and 3 for both alleles ( the nucleus is representative of 116 imaged nuclei of pluripotent stem cells; upper panels). Alleles of chromosomes 1 and 3 were separated in mesendodermal OCT4-OE cells (the nucleus is representative of 110 nuclei; lower panels). The red, green channels and the merged image are shown. Scale bar, 2 μm. The probe hybridized region is magnified in the inset of the merged image. The right graph in the inset indicates the averaged percentage of cells featuring aSox-2/Sox-17interaction from three experiments (*Student’st-test,P≤0.01). Figure 7: OCT4 breaks Sox-2/Sox-17 enhancer inter-chromosomal interaction. ( a ) 3C experiments were performed on digested and religated chromatin from undifferentiated ZHBTc6 cells or OCT4-induced mesendodermal cells. Primers spanning within the Sox-2 and Sox-17 loci and numbered as in Table 2 were used in PCR. Control primers, such as in exons, were used as controls (cartoons, a – c ). Interaction frequencies were normalized using the GAPDH locus. The graphs show the frequency of interactions between chromosomes (Chr) 1 and 3. The gels show the specificity of the amplicons of the peaks of interaction; the sequence of amplicons was checked by sequencing. The relative interaction frequency value is set to one for the interaction measured between the control GAPDH fragments. Data are representative of four experiments (mean±s.e.m.). ( b ) Illustration of FISH experiments using a Sox2 alexa488 and Sox17 alexa568 probes showing the interaction between chromosomes 1 and 3 for both alleles ( the nucleus is representative of 116 imaged nuclei of pluripotent stem cells; upper panels). Alleles of chromosomes 1 and 3 were separated in mesendodermal OCT4-OE cells (the nucleus is representative of 110 nuclei; lower panels). The red, green channels and the merged image are shown. Scale bar, 2 μm. The probe hybridized region is magnified in the inset of the merged image. The right graph in the inset indicates the averaged percentage of cells featuring a Sox-2/Sox-17 interaction from three experiments (*Student’s t -test, P ≤0.01). Full size image Cohesin loading is required for OCT4-induced cardiogenesis Our previous findings pointed to a key role of the cohesin complex in mediating OCT4-induced changes in higher-order chromatin structure at Sox loci. NIPBL was downregulated using a siRNA as described in Fig. 5 . Two days following cell transfection with siRNA, OCT4 expression was induced by washing out tetracycline from ZHBTc6 cell culture medium and EBs were generated using the hanging drop protocol [15] . Day 7 EBs featured expression of cardiac markers such as Nkx2.5 , Mef2c , Isl1 , Tbx5 or cardiac α-actin , which were significantly increased in EBs formed from OCT4-overexpressing cells. EBs generated from NIPBL-downregulated ZHBTc6 cells in which OCT4 was upregulated featured a more modest increase in cardiac-enriched genes than mock EBs fully expressing NIPBL generated from mock ESC transfected with a random sequence siRNA ( Fig. 8a ). The blunted OCT4-induced cardiac transcriptional response by a reduction in NIPBL was translated into a decrease in the process of cardiac differentiation as shown by a decrease in Nkx2.5 + (22±5% of total nuclei/field in OCT4OE mock versus 9±2% in siRNA NIPBL-downregulated cell), Isl1 + (34±8% of total nuclei/field in OCT4OE versus 14±5% in siRNA NIPBL downregulated cell) and actinin + cells (18±7% of total cells/field in OCT4OE versus 3±2% in siRNA NIPBL-downregulated cells), as well as a mislocation of Nkx2.5 in the cytosol of cells in contrast to the nuclear location in mock cells ( Fig. 8b ). Expression of ectodermal-enriched genes such as Nestin, Ck17 or Pax3 , as well as endodermal genes such as Foxa2 , HFN4 or albumin , was not affected by OCT4 overexpression or by the absence of NIPBL ( Fig. 8c ). 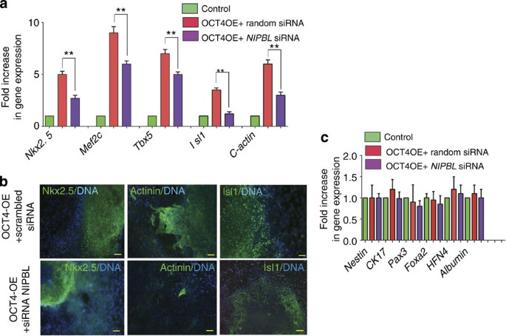Figure 8: NIPBL-mediated loading of the cohesin complex is required for the cardiogenic effect of OCT4. NIBPL was downregulated by a siRNA. Cardiogenesis was monitored by the gene expression of cardiac-enriched genes (a) and (b) by immunostaining of cardiac transcription factors Nkx2.5 and Isl1 and a sarcomeric protein (actinin) in day 12 EBs. Scale bar indicates 50 μm. (c) Ectodermal and endodermal genes were monitored. Data are representative of three experiments (mean±s.e.m., *Student’st-test,P≤0.01). Figure 8: NIPBL-mediated loading of the cohesin complex is required for the cardiogenic effect of OCT4. NIBPL was downregulated by a siRNA. Cardiogenesis was monitored by the gene expression of cardiac-enriched genes ( a ) and ( b ) by immunostaining of cardiac transcription factors Nkx2.5 and Isl1 and a sarcomeric protein (actinin) in day 12 EBs. Scale bar indicates 50 μm. ( c ) Ectodermal and endodermal genes were monitored. Data are representative of three experiments (mean±s.e.m., *Student’s t -test, P ≤0.01). Full size image Our findings show that the OCT4/SALL4 duo is a key complex of transcription factors acting in a gene dosage-dependent manner to remodel chromatin architecture around the Sox-2/Sox-17 loci and to switch embryonic cell fate from epiblast towards the cardiogenic mesoderm. A twofold increase in OCT4 protein in ESCs allowed us to recapitulate an early step of embryonic development by giving rise to a mesendodermal cell population ( Fig. 2 ). Genome-wide ChIP analysis of OCT4 target sites in mesendodermal cells, although investigating only the binding sites closest to the gene transcription starting sites (that is, within 10-kb range) together with sequential ChIP assays and its co-expression with OCT4 in E7.5 embryos, uncovered SALL4 as a privileged target and partner of the POU factor in mesendodermal cells. Both the OCT4 and SALL4 transcription factors act together as triggers of changes in chromatin architecture to switch the fate of embryonic cells from pluripotency to that of cardiac progenitors. This event revealed a major and combined role of the cohesin and polycomb complexes in cell fate decision. A recent pioneering publication showed that a change in the topological structure of chromatin, including mainly long-range DNA interaction, occurs when stem cells differentiate towards a neuronal progeny [12] . We now extend this concept to the dynamics of short-range interactions within topological domains [10] , which also concur to cell fate decisions and we provide a mechanistic explanation for such molecular events at specific Sox loci. We localized OCT4 by whole-mount staining of mouse late streak embryo, co-expressed with SOX-17 and SALL4 in the visceral endoderm and in the mesendoderm. The latter segregates into endoderm and mesoderm, which patterns into the LPM among others. OCT4 then gives rise within the LPM to MesP1 + cardiovascular progenitors ( Fig. 1 ). These findings further document the observation of Downs [38] and highlight the biological relevance of OCT4 binding to MesP1 + regulatory regions [19] . Our data show that OCT4 acts as a cardiac instructor through its indirect action within the BMP2-secreting visceral endoderm [39] , and through a direct effect within the mesendoderm, and derived EOMES + and MESP1 + mesoderm, both genes being turned on following Nodal- and BMP-induced OCT4 upregulation [15] , [40] , [41] . SALL4 is upregulated in OCT4-overexpressing mesendodermal cells and in turn is likely to target new genes in the later cells as previously shown in Xen cells [21] . It is a protein required for the OCT4-triggered changes in chromatin architecture at Sox loci and in turn the cardiogenic functions of OCT4, and thus plays a crucial role in early development. SALL4 is first expressed in extraembryonic visceral endoderm [42] ( Fig. 1 ), and is cell autonomously required for the development of the epiblast and primitive endoderm from the inner cell mass [43] . Tetraploid rescue of SALL4 knockout embryos further revealed a requirement in Wnt/beta-catenin signalling to effect antero-posterior (AP) axis elongation during gastrulation. SALL4 expression is mandatory within the early embryo to initiate BMP expression in extraembryonic endoderm and Nodal expression in epiblast, two pathways regulating OCT4 and early mesoderm formation [42] . SALL4 is also regulated by Wnt3 (ref. 44 ), an inducer of mesendoderm [45] , and a factor secreted from OCT4-induced SOX-17 + cells [16] . SALL4 null mutant mice die shortly after implantation, which can be explained by the role of SALL4 in early embryogenesis, as we and others [41] have reported. SALL4 haploinsufficiency leads, among other defects, to heart abnormalities [31] as expected from its role in early cardiogenesis. Finally, SALL4 plays a key role in recruiting the polycomb complex (both PRC1 and PRC2) to the Sox-2 promoter and enhancer to silence the transcription of this gene ( Fig. 4 ) and in turn to change the epigenetic marks, including H3K27me3, on Sox regulatory regions ( Supplementary Fig. 2 ). Importantly, the recruitment of polycombs might also participate in breaking the Sox-2C and Sox-17 enhancer interaction by targeting the Sox-2 locus to polycomb bodies [46] . Interestingly, PCR1 and PRC2 occupation of the Sox-17 l ocus in pluripotent cells is lost in a SALL4-dependent manner when cells are committed to the mesendodermal cell fate ( Fig. 3 ). It should, however, be noted that PRC1 alone remains on the Sox-17 promoter and even increases on Sox-17 enhancer, while the gene is transcriptionally active thanks to the cohesin-dependent loop formed between the enhancer and promoter ( Fig. 4 ). Thus, PRC1 alone might play together with cohesin an active role in the formation or maintenance of chromatin loops and gene transcription as recently proposed [47] , [48] . The most striking and original finding in our study is the manner by which OCT4 acts on the cohesin complex to disrupt an inter-chromosomal SOX-2/SOX-17 CTCF-dependent interaction that prevents the 3′- SOX-17 enhancer from folding onto its own promoter. OCT4- and SALL4-mediated chromatin-remodelling allows for the relief of this inhibition, and an activation of the SOX-17 promoter following the formation of a cohesin-dependent enhancer-promoter loop and trimethylation of H3K4 on the SOX-17 locus ( Figs 4 , 6 , 7 ; Supplementary Fig. 2 ). A downregulation of NIPBL, as seen in the Cornelia de Lange syndrome, prevented the switch of OCT4 from Sox-2c to Sox-17 enhancers ( Fig. 5 ) and significantly affected cardiogenesis induced by OCT4 ( Fig. 8 ), indicating that a cohesin-mediated change in higher-order chromatin structure at the Sox loci is required for cardiogenesis. Our data further document that CTCF-independent cohesin binding to tissue-specific transcriptions factors regulatory regions of genes such as Sox-2 and Sox-17 , is highly cell-type specific. Cohesin might favour the stabilization of OCT4 on the Sox-17 locus [49] . Furthermore, our findings argue for the first time in favour of enhancers (that is, Sox-2 ) playing the role of both activator on gene promoters (within intra-chromosomal interactions) and repressor by sequestering another enhancer (that is, Sox-17 ) within an inter-chromosomal interaction. In the same line of thinking, promoter interactions with specific enhancers are finely tuned in specific cell types at specific developmental stages. As another example, OCT4 and SOX-17 both specifically bind to a compressed non-canonical enhancer in endodermal cells [50] , in contrast to mesendodermal and mesodermal cells in which they bind to canonical octamer sites. Interestingly, the chromosomes 3 and 8 in human cells harbouring Sox-2 and Sox-17 , respectively, are localized to the same chromosomal territory [51] . In a broader view, our data further suggest that the formation of specific DNA–DNA interactions within pre-existing chromatin territories is likely to be cell specific and to change during the development [49] . Using mouse embryos, HUESCs and mouse ESCs, powerful models of early development, we have delineated a mechanistic pathway that underlies the OCT4/SALL4 auto-regulatory cardiogenic loop, and the specific function of SALL4 in early cell fate decisions in the embryo. SALL4, a new partner of OCT4 in its function of cell fate determination, serves as a recruiting factor to facilitate the switch of OCT4 from Sox-2 to Sox-17 enhancers, by directing the targeting of histone modifiers such as polycombs, which altogether drive embryonic cells towards a mesendodermal and cardiac fate. This switch is driven by the cohesin-mediated chromatin-remodelling concomitantly triggered by OCT4 ( Fig. 9 ). 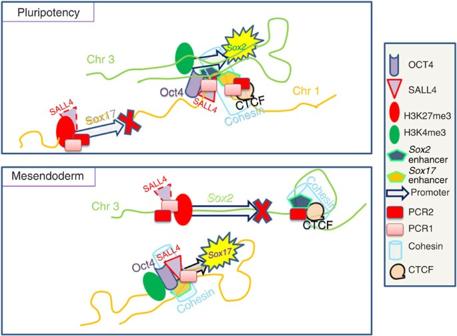Figure 9: Mechanistic model of OCT4/SALL4 changes in higher-order chromatin structure. Cartoon illustrating the inter- and intra-chromosomal interactions within theSox-2andSox-17loci, as well as the location of bivalent epigenetic marks and polycomb complexes in pluripotent (inner cell mass (ICM)-like cells) and mesendodermal cells. Figure 9: Mechanistic model of OCT4/SALL4 changes in higher-order chromatin structure. Cartoon illustrating the inter- and intra-chromosomal interactions within the Sox-2 and Sox-17 loci, as well as the location of bivalent epigenetic marks and polycomb complexes in pluripotent (inner cell mass (ICM)-like cells) and mesendodermal cells. Full size image Our findings further revealed a SALL4/OCT4 complex as a primary cardiac inducer. Defects in this early pathway following the mutation of one of these factors, or a defect in formation of their associated chromatin or nucleosome remodelers, might be at the crossroads of congenital cardiac diseases involving SALL4, as in Okihiro syndrome [52] , or both SALL4 and the cardiac transcription factor NKX2.5, as in the Wolf–Hirschhorn syndrome [53] . Our data offer a possible explanation for cardiac defects in Cornelia de Lange syndrome caused by mutations in cohesin-loading factors, as well as proteins of the cohesin complex, which are characterized by severe developmental defects. In this syndrome, recently modelled in zebrafish, the SOX-17-EOMES pathway is severely affected [54] as predicted by our current findings. Our findings provide evidence that although both stemness (OCT4, SOX-2 and SALL4) and differentiation (SOX-17, SALL4, ISL1, NKX2.5 and TBX5) gene modules exist [55] , the same transcription factors can switch from one to the other module and combine with new binding partners (OCT4/SOX-2/SOX-17) to coordinate and orchestrate early cell fate decisions, and cell differentiation. Such a phenomenon requires a change in the higher-order chromatin structure. OCT4, which accesses the Sox-17 locus by targeting the cohesin complex as well as many chromatin remodelling enzymes, might be considered as a pioneer factor [56] , which drives the pluripotent cells towards a cardiogenic cell fate. The role of OCT4 could be further facilitated by the action of cohesins as nucleosome repositioning agents [57] . Mice Embryos were staged as E0.5 the day of observation of the vaginal plug. MesP1Cre mice were obtained originally from Dr Saga and were kindly given by Dr R Kelly’s laboratory (IBDM, CNRS Luminy Marseille). These mice were genotyped using Cre primers (forward 5′-AGTTGCTTCAAAAATCCCTTCCAGGGCCCG-3′ and reverse 5′-AGCAATGCTGTTTCACTGGTTATGCGGCGG-3′). 129S6-Gt(ROSA)26Sortm9(CAG-dTomato)Hze/J were obtained from The Jackson laboratory and genotyped using for wild-type allele: forward 5′-AAGGGAGCTGCAGTGGAGTA-3′ and reverse 5′-CCGAAAATCTGTGGGAAGTC-3′, mutant forward 5′-GGCATTAAAGCAGCGTACC-3′ and reverse 5′-CTGTTCCTGTACGGCATGG-3′. The Sox17Cre mouse was obtained from The Jackson laboratory and genotyped using Cre primers as described above. Mice experiments were performed in agreement with a local ethical committee and following the Animal health and welfare guide lines of the European Union. Embryos whole-mount staining Whole-mount staining of embryos was performed as already published by Dr Janet Rossant’s laboratory. Briefly, embryos were fixed overnight at 4 °C with 4% paraformaldehyde, washed with PBS Triton X100 0.1%, permeabilised with PBS Triton 0.25% and blocked with PBS 0.1% Triton X100 added with 10% FCS; the first antibody was added in PBS 10% FCS and 1% Triton X100. The second antibody was added in PBS 0.1% Triton X100. The antibodies used were anti-OCT4 (sc-9181), anti-SOX-17 (R&D AF1924) and anti-SALL4 (sc-46045) used at 1/100 and were all already used in the literature (list available on request) and shown to be specific. Alexa-conjugated antibodies (1/400; Life Technologies, France) were used as secondary antibodies. Control immunostaining were performed on embryos using only the secondary antibodies. Specificity was further checked in this study in cells lacking the expression of the proteins (knocked down ESCs, mouse embryonic fibroblasts (MEF)) both in western blotting and ChIP, as well as immunofluorescence. Embryos were imaged in confocal microscopy. Stacks of images were acquired and used to reconstruct the embryo using AMIRA software (VSG). Cardiac commitment of human pluripotent stem cells Two HUESC lines, that is, HUES-24 and HUES-9 pOct4/green fluorescent protein (GFP), were used throughout this study without any difference in the data. HUESCs were cultured on mouse embryonic fibroblasts from E14 Mouse embryos, using KO-DMEM medium supplemented with β-mercaptoethanol, glutamine, non-essential amino acids, 15% knock-out serum replacement (KOSR) and 10 ng ml −1 fibroblast growth factor 2 (FGF2). Medium was changed every day. Cell colonies were dissociated into single cells every 4 days using trypsin. Cell nucleofection with OCT4-iA was performed with AMAXA kit according to the manufacturer. The cells were then plated on matrigel-coated dishes in HUESCs MEF-conditioned medium supplemented with FGF2 for 4 days to reach a twofold increase in the OCT4 protein level. Cells were phenotyped every 10 passages using anti-SSEA-3/4, TRA-1-60 and TRA-1-80 antibodies used at 1/100 (Chemicon kit SCR-002). Less than 5% of cells were positive for SSEA-1 (Chemicon). Karyotype was found normal and stable in the course of the experiments. EBs were generated from mock pcDNA nucleofected or Oct4-iA-nucleofected HUESCs 4 days post nucleofection in DMEM added with 20% FCS. Cells were let in suspension for 6 days to allow for their aggregation and then EBs were dissociated with trypsin and plated on cells plated for 14 h on fibronectin-coated labtech plates. Culture of ZHBTc6 mouse ESCs Mouse ESCs were cultured and OCT4 was induced as previously described [15] . To avoid any leakage of the Tc-regulated transgene, and to ensure a precise increase in OCT4 when tetracycline is removed, the ZHBTc6 parental cell line kindly given by Dr Niwa was subcloned and three different selected subclones were used in the study without significant differences in data obtained with these cell lines. Removal of tetracycline led to a twofold increase in OCT4 protein. 3D FISH . Amplicons (1.2 Kb) including Sox-2C and Sox-17 enhancers were amplified by PCR from bacterial artificial chromosoma (BACS) and were labelled with ChromaTide Alexa Fluor 488-5 dUTP and ChromaTide Alexa Fluor 568-5 dUTP (Life Technologies), respectively, by Nick translation. The FISH protocol was adapted from ref. 58 . Mouse ESC cultured on gelatine-coated labtech dishes were fixed with 4% paraformaldehyde for 10 min, washed with PBS and permeabilized with 0.5% Triton X100 for 30 min. Cells were washed with PBS, PBS/20% glycerol and frozen overnight at −20 °C in PBS/50% glycerol. The next day, cells were further permeabilized by six freeze-thaw cycles in liquid nitrogen. Denaturation of proteins was performed using 0.1 N HCl for 30 min, and the cells were stored for 5 days in 50% formamide/50% SSC 2 × at 4 °C. Cells were then hybridized using 10 μl mix including hybridation solution B (Cytocell), DNA-coat and the DNA-alexa Sox-2 and Sox-17 probes (0.3–1 ng) spotted on a coverslip put on cells and fixed with rubber cement. The cells and probes were concomitantly denatured for 2 min on a hot plate (78 °C) and incubated overnight at 37 °C. Cells were then thoroughly washed with 0.2 × and 1 × SSC buffer at 63 and 45 °C, and counterstained with 5 μg ml −1 4,6-diamidino-2-phenylindole. At least 110 cells in each experimental condition (control or OCT4OE cells) were monitored in three separate experiments. Image stacks were taken at 0.5 μm steps from cells and processed using Image J. Images from stacks were projected onto one plane. Real-time quantitative PCR RNA was extracted from ESCs using a Zymo Research (Orange, CA, USA, Proteingene, France) kit. One microgram of RNA was reverse transcribed using the SuperscriptII reverse transcriptase (Invitrogen, Cergy, France) and oligo(16)dT. Quantitative PCR was performed using a Light Cycler LC 1.5(Roche Diagnostic). Amplification was carried out as recommended by the manufacturer. Twelve microlitre reaction mixture contained 10 μl of Roche SYBR Green I mix, respectively (including Taq DNA polymerase, reaction buffer, deoxynucleoside trisphosphate mix, SYBR Green I dye and 3 mM MgCl 2 ), 0.25-μM concentration of appropriate primer and 2 μl of diluted complementary DNA (cDNA). The amplification programme included the initial denaturation step at 95 °C for 8 min, and 40–60 cycles of denaturation at 95 °C, annealing at 65 °C for 8 s and extension at 72 °C for 10 s. The temperature transition rate was 20 °C s −1 . Fluorescence was measured at the end of each extension step. After amplification, a melting curve was acquired by heating the product at 20 °C s −1 to 95 °C, cooling it at 20 °C s −1 to 70 °C, keeping it at 70 °C for 20 s and then slowly heating it at 20 °C s −1 to 95 °C. Fluorescence was measured through the slow heating phase. Melting curves were used to determine the specificity of PCR products, which were confirmed using conventional gel electrophoresis and sequencing. Data were analysed according to Pfaffl [59] . Primers specific for human genes are described in ref. 60 and include MIXL1 , forward: 5′-TCTTCCGACAGACCATGTACC and reverse 5′-TTCTGGAACCACACCTGGAT-3′; SPARC, forward 5′-AAGATCCATGAGAATGACAAG-3′ and reverse: 5′-AAAAGCGGGTGGTGCAATG-3′; NOGGIN , forward 5′-CCATCATTTCCGAGTGCAAGTGCT-3′ and reverse 5′-AAGCTAGGTCTCTGTAGCCCAGAA-3′; and PAX6 , forward 5′-AGTGAATCAGCTCGGTGGTGTCTT-3′ and reverse 5′-TGCAGAATTCGGGAAATGTCGCAC-3′. Chromatin immunoprecipitation assay ChIP was performed according to a standard ChIP protocol [15] or the Fast ChIP protocol [61] . The ChIP grade antibodies used were anti-OCT4 (Santa Cruz; sc-9081 and sc-5279), anti-SALL4 (Santa Cruz; sc-46046 raised against 200 amino acids of N-terminal domain), anti-CTCF and –RAD21 (references 07–729 and 05–908, respectively, Millipore, France), anti-SUZ12 (CS-029-050; Diagenode) anti H3K4me3 (C15410003-50; Diagenode) and antiH3K27me3 (C15410195; Diagenode), anti-BMI1 (Abcam; ab-14389). All antibodies used at 1 μg per 100 μg chromatin have been validated in preliminary ChIP experiments, as well as in previous publications (list available on request). Absolute enrichment was calculated assuming that at most 1% of nucleosome was immunoprecipitated [62] . Genomic region was thus considered enriched if 10-ng immunopricipitated samples showed a greater enrichment when compared with 0.1 ng of input DNA. Results are expressed as percentages of the input. For the sequential ChIP experiments (double ChIP), proteins–DNA complexes after the first anti-OCT4 or SALL4 ChIP were extensively washed with ChIP buffer and then a Tris-EDTA buffer. Complexes were eluted by incubation for 30 min at 37 °C in 50 μl of elution buffer TE buffer supplemented with 2% SDS, 15 mM dithiothreitol and protease inhibitors. This reducing protocol cleaves the antibody so that no trace of first antibody remains during the second immunoprecipitation reaction. After centrifugation, the supernatant was diluted 20 times with ChIP buffer and the samples were then subjected to the ChIP protocol. The primers used to amplify the genomic regions of enhancers and promoters are listed in Supplementary Table 1 . Control immunoprecipitation (mock) were performed using control IgG or no antibody with similar results. Sizes of PCR amplicons were checked on gels and products sequenced. ChIP on chip ChIP was performed as described above. The pulled down DNA was amplified and hybridized to Affymetrix—GeneChip Human Promoter 1.0R tiling Array according to the manufacturer. The array includes 4.6 million probes tiled through over 25,500 human promoter/enhancer regions. Experiments were performed in duplicate of biological samples. To identify OCT4 target sites, we compared the ChIP-chip intensities of the HUESCs nucleofected with OCT4-iA cDNA to those of GFP-nuclected HUESCs. Before the binding site detection, raw intensity data were normalized between the controls and the corresponding Oct4iAOE cells using the cross-correlation method [63] . Enriched binding sites were identified based on peak height intensity, peak weight and peak neighbouring intensities. To ensure that the identified binding sites is enriched, statistical distributions of log2 fold changes of the enriched binding sites is compared with the distribution of background noise and 5% false discovery rate is used to select enriched binding sites. The identified binding sites were then mapped to the gene promoter sites that are available from Genomatrix ( http://www.genomatix.de ). Only those enriched ChIP-chip binding sites that were overlapped with the promoter sites were recognized as genes targeted by OCT4-iA. Peak and non-peak visualization was carried out with a NimbleGen genome viewer. 3C experiments 3C experiments were performed and analysed according to Naumova et al. [64] Briefly, ESCs were crosslinked with 1% formaldehyde for 10 min and quenched with 125 mM glycine. The cells were then permeabilised and lysed using the ChIP buffers to get the nuclear fraction [15] . Chromatin was digested by DpnII. The digestion was monitored by specific primers spanning DpnII sites in the genome Supplementary Table 2 . Chromatin was diluted and digested fragments ligated overnight in the T4 ligase buffer. DNA was extracted by phenol/chloroform and used in real-time PCR. Amplicons were run on gel and sequenced. Bacterial artificial chromosoma clones spanning the Sox-2 and Sox-17 loci were obtained from the Sanger Bank (RPCI-23-37D15 and RPCI-23-129D12) spanning the Sox-17 or the Sox-2 locus, respectively, were used as linear DNA undigested or digested with DpnII and religated as a control template library for 3C primers. All primers were designed or re-designed to feature the same efficiency. 3C primers including control primers and the glyceraldehyde 3-phosphate dehydrogenase (GAPDH) site primers used are listed in Supplementary Table 2 . The relative interaction frequency for a given primer pair is calculated by the ratio of the amount of PCR amplicon of the samples corrected with the control region, previously checked as a non-interactive regions ( Sox-17 TSS+110 kb, or Sox-2 3′-TSS+20 kb) versus the control template. Normalization was done using the ligation product of a control fragment in the GAPDH locus. GAPDH being a housekeeping gene expressed to the same extent in both pluripotent stem cells and OCT4OE mesendodermal cells, the 3D configuration of the locus was assumed to be unchanged. Data are an average of four biological replicates, each run twice in PCR. All DNAs were measured using SYBGR and a standard curve prepared from input DNA. DNA constructs Human SALL4 ShRNA sequences (5′-gatcccctcatttgccaccgagtcttttcaagagaaagactcggtggcaaatgatttttc-3′) was synthesised as a sense and antisense oligonucleotide, annealed and subcloned in the pSuper vector (Ambion). The DNA construct was nucleofected in Human ESCs, using Amaxa-specific nucleofector solution I, as recommended by the manufacturer. A scramble Sh cloned in the pSuper vector targeting a random sequence (5′-agacagcgatcgtcttctcttgcccgcggagagaacagtttcgctgtcttttttt-β) was used as a control. OCT4-iA was amplified from RNA extracted from HUESCs as described in ref. 16 and subcloned in a pcDNA vector. Mouse Sall4 siRNA (esiRNA) was from SIGMA, France; mouse NIPBL siRNA was from Santa Cruz. Scrambled siRNAs were designed by generating random sequences and used as controls in mock cells. Cell immunofluorescence Cell immunofluorescence was carried out as previously described [15] . The anti-SOX-17 antibody was from R&D (Mab1924). The anti-SALL4 was from Santa Cruz (sc-46045); the anti-NIPBL antibody was from Abbiotec (#25013) and used at 1/100 dilution. Protein immunoprecipitation and western blots Cells were nucleofected with OCT4-iA cDNA or backbone pcDNA using the kit V (Amaxa). Chromatin was then extracted 2 days later according to the ChIP protocol described above. Co-Immunoprecipitation was performed in radio-immunoprecipitation assay (RIPA) buffer and western blot analysis was conducted as previously reported [16] . The anti-OCT4 antibodies used were from Santa Cruz (N19 and H-134). Normalization of blots was performed using an anti-actin antibody (Sigma-Aldrich A2066 used at 1/1,000). Quantification of bands was carried out using Quanti one software (BioRad). SALL4 and OCT4 western blots were performed using the anti-SALL4 from Abcam (ab29112) and anti-OCT4 (H-134) antibody recognizing both OCT4-iA and iB and anti-RAD21 antibody (05–908 Millipore) all used at 1/1,000 dilution. Accession codes: ChIP-chip data have been deposited in the NCBI Gene Expression Omnibus under accession code GSE58125 . How to cite this article: Abboud, N. et al. A cohesin–OCT4 complex mediates Sox enhancers to prime an early embryonic lineage. Nat. Commun. 6:6749 doi: 10.1038/ncomms7749 (2015).